Cdk5 controls lymphatic vessel development and function by phosphorylation of Foxc2 The lymphatic system maintains tissue fluid balance, and dysfunction of lymphatic vessels and valves causes human lymphedema syndromes. Yet, our knowledge of the molecular mechanisms underlying lymphatic vessel development is still limited. Here, we show that cyclin-dependent kinase 5 (Cdk5) is an essential regulator of lymphatic vessel development. Endothelial-specific Cdk5 knockdown causes congenital lymphatic dysfunction and lymphedema due to defective lymphatic vessel patterning and valve formation. We identify the transcription factor Foxc2 as a key substrate of Cdk5 in the lymphatic vasculature, mechanistically linking Cdk5 to lymphatic development and valve morphogenesis. Collectively, our findings show that Cdk5–Foxc2 interaction represents a critical regulator of lymphatic vessel development and the transcriptional network underlying lymphatic vascular remodeling. The lymphatic system maintains key physiological functions like tissue fluid homeostasis, immune surveillance and uptake of dietary lipids. In consequence, the lymphatic vasculature plays a key role in various human pathologies. Lymphangiogenesis occurs in chronic inflammation and tumour dissemination, and dysfunction of lymphatic vessels causes human lymphedema syndromes [1] . Yet, our knowledge about the mechanisms regulating lymphatic vessel development and function is still limited. Lymphatic vessel formation starts after the circulatory system is established. Lymphatic endothelial cells emerge from the cardinal veins and migrate away to form the primary lymphatic vessels, that is, the lymph sacs, which get separated from the blood vasculature by lymphovenous valves [2] , [3] , [4] . Peripheral lymphatic vessels remodel into lymphatic capillaries that take up interstitial fluid and collecting lymphatic vessels that drain the lymph into the venous system. Lymphatic capillaries are blind-ending and lack mural cells, whereas collecting lymphatic vessels contain smooth muscle cell (SMC) coverage and intraluminal valves [5] . Several regulators of lymphatic vessel remodelling and valve formation have been identified, including ephrinB2 (ref. 6 ), integrin-α9 (ref. 7 ), semaphorinA3 (refs 8 , 9 ), Prox1 (ref. 4 ) and Foxc2 (ref. 10 ). Yet, their molecular regulation in the lymphatic endothelium is largely unknown. Cyclin-dependent kinase 5 (Cdk5), a proline-directed serine/threonine kinase, does not drive cell cycle transitions though it belongs to the Cdk family. As it exerts essential functions in the central nervous system (CNS) such as neuronal migration, axonal guidance and synaptic plasticity, and has been associated with neurodegenerative and neuropsychiatric diseases, Cdk5 was thought to be neuron-specific for a long time [11] . Recently, awareness about extra-neuronal functions of Cdk5 has grown. Cdk5 was linked with inflammation, that is, leukocyte activation, with obesity and insulin resistance by phosphorylating the transcription factor PPARγ, and some reports indicate functions of Cdk5 in cancer (reviewed in ref. 12 ). In contrast, a detailed investigation of a possible function of Cdk5 in the endothelium in vivo is still lacking. To address this issue, we generated two endothelial-specific Cdk5 knockout models to study the mechanism of action of Cdk5 in the vascular system, including the search for the functionally relevant endothelial substrate of Cdk5. We show that Cdk5 plays an essential role in the regulation of lymphatic vessel development and valve formation. Mechanistically, we demonstrate that Cdk5 phosphorylates and regulates the activity of the transcription factor Foxc2. This mechanism contributes to the poorly understood regulation of Foxc2 in lymphatic vessel development and reveals an unexpected role of Cdk5 in the lymphatic vasculature. Phenotype of endothelial-specific Cdk5 knockout mice Cdk5 and its activator p35 are ubiquitously expressed in the vasculature ( Supplementary Figs 1 and 2 ). We disrupted the Cdk5 gene specifically in the mouse endothelium by using the Cre/loxP system with a constitutive Tie2Cre and a tamoxifen-inducible VE-Cadherin Cdh5(PAC)-CreERT2 transgene [13] ( Supplementary Figs 2 and 3 ). Loss of Cdk5 in the mouse endothelium resulted in postnatal lethality with >40% of mice dying during the first 2 days after birth or at the age of 3–4 weeks after weaning ( Fig. 1a ). Born Cdk5 fl/fl Tie2Cre mice showed reduced size and body weight ( Fig. 1b,c ) and we observed frequent bleedings ( Fig. 1d , Supplementary Fig. 2e ). Instead of expected 25%, only 15% of progeny had the Cdk5 fl/fl Tie2Cre genotype ( Fig. 1e ), suggesting embryonic lethality. Indeed, endothelial-specific Cdk5 knockout embryos died from E16.5 onwards. They showed blood-filled dilated tortuous vessels extending from the jugular region towards the abdominal area, bleedings, especially prevalent in jugular regions and edema formation ( Fig. 1f–h ), indicating severe lymphatic vessel defects. Cdk5 protein levels were attenuated in lymphatic endothelial cells (LECs) and blood vessel endothelial cells (BECs) of Cdk5 fl/fl Tie2Cre embryos ( Fig. 1i ). Identity and purity of isolated LECs and BECs were confirmed by immunostainings that show expression of Prox1 and VEGFR3 in LECs, but not in BECs, in the macrophage/leukocyte fraction nor in residual cells ( Supplementary Fig. 4 ). The Tie2 promoter is active both in endothelial cells and some hematopoietic cells such as monocytes or macrophages [14] . In addition, functions of Cdk5 in the hematopoietic system have been reported, including an implication of Cdk5 in T-cell activation and experimental autoimmune encephalomyelitis [15] or an involvement of Cdk5 in hematopoietic cell differentiation [16] , [17] , [18] . To confirm the role of Cdk5 in endothelial cells, we used a VE-Cadherin (VEC) Cre driver line, that is, the tamoxifen-inducible Cdh5(PAC)-CreERT2 line. Cdk5 fl/fl Cdh5(PAC) – CreERT2 (Cdk5 fl/fl VECCre) embryos from tamoxifen-treated mothers show a highly similar phenotype as embryos with Cdk5 fl/fl Tie2Cre genotype ( Fig. 1f,g ), demonstrating an endothelial cell autonomous function of Cdk5. To assess the effect of more prevalent loss of Cdk5 in the endothelium, we derived mice in which one Cdk5 allele was constitutively deleted (Δ) and the remaining allele was floxed (fl) ( Fig. 1h,j ). Indeed, embryos with Cdk5 Δ /fl Tie2Cre genotype died at E15.5, with blood-filled dilated tortuous vessels, hemorrhaging and edema formation ( Fig. 1h ). Thus, more pronounced loss of Cdk5 resulted in more severe lymphatic deficiencies. In summary, the similarity of the phenotypes of endothelial Cdk5 knockdown mice achieved by different Cre driver lines indicates a specific and essential function of endothelial Cdk5 for lymphatic vessel development. 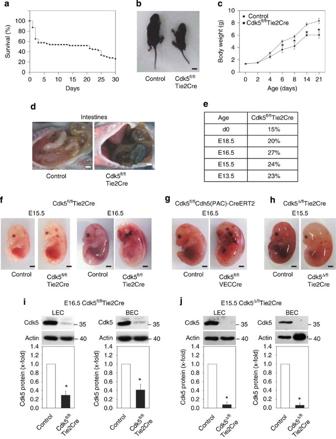Figure 1: Endothelial cell-specific Cdk5 knockout mice. (a) Impaired survival ofCdk5fl/flTie2Cremice. The Kaplan–Meier plot indicates that 40%Cdk5fl/flTie2Cremice died during the first 2 days, 75% during the first 30 days after birth; 352 mice; 54Cdk5fl/flTie2Cremice. (b) Reduced size ofCdk5fl/flTie2Cremice (d11). Scale bar, 2 cm. (c) Reduced body weight ofCdk5fl/flTie2Cremice.t-test, *P≤0.05, s.e.m.;n≥4 per age and genotype. (d) Intestinal bleeding ofCdk5fl/flTie2Cremice (d20). Scale bar, 1 cm. (e) Embryonic lethality ofCdk5fl/flTie2Creembryos. Percent of livingCdk5fl/flTie2Creembryos at indicated stages. (f–h) Blood-filled leaky superficial capillaries, bleeding and edema formation in EC-specific Cdk5 knockout embryos. (f) E15.5 and E16.5Cdk5fl/flTie2Creembryos. Scale bar, 2 mm. (g) E16.5Cdk5fl/flVECCreembryos. Scale bar, 2 mm. (h) E15.5Cdk5Δ/flTie2Creembryos. Scale bar, 2 mm. (i) Decreased Cdk5 levels in LECs (29%) and BECs (41%) of E16.5Cdk5fl/flTie2Creembryos. Each:t-test, *P≤0.001, s.e.m.;n=8 per genotype. (j) Decreased Cdk5 levels in LECs (7.8%) and BECs (6.4%) of E15.5Cdk5Δ/flTie2Creembryos. Each:t-test, *P≤0.001, s.e.m.;n=3 per genotype. Figure 1: Endothelial cell-specific Cdk5 knockout mice. ( a ) Impaired survival of Cdk5 fl/fl Tie2Cre mice. The Kaplan–Meier plot indicates that 40% Cdk5 fl/fl Tie2Cre mice died during the first 2 days, 75% during the first 30 days after birth; 352 mice; 54 Cdk5 fl/fl Tie2Cre mice. ( b ) Reduced size of Cdk5 fl/fl Tie2Cre mice (d11). Scale bar, 2 cm. ( c ) Reduced body weight of Cdk5 fl/fl Tie2Cre mice. t -test, * P ≤0.05, s.e.m. ; n ≥4 per age and genotype. ( d ) Intestinal bleeding of Cdk5 fl/fl Tie2Cre mice (d20). Scale bar, 1 cm. ( e ) Embryonic lethality of Cdk5 fl/fl Tie2Cre embryos. Percent of living Cdk5 fl/fl Tie2Cre embryos at indicated stages. ( f – h ) Blood-filled leaky superficial capillaries, bleeding and edema formation in EC-specific Cdk5 knockout embryos. ( f ) E15.5 and E16.5 Cdk5 fl/fl Tie2Cre embryos. Scale bar, 2 mm. ( g ) E16.5 Cdk5 fl/fl VECCre embryos. Scale bar, 2 mm. ( h ) E15.5 Cdk5 Δ /fl Tie2Cre embryos. Scale bar, 2 mm. ( i ) Decreased Cdk5 levels in LECs (29%) and BECs (41%) of E16.5 Cdk5 fl/fl Tie2Cre embryos. Each: t -test, * P ≤0.001, s.e.m. ; n =8 per genotype. ( j ) Decreased Cdk5 levels in LECs (7.8%) and BECs (6.4%) of E15.5 Cdk5 Δ /fl Tie2Cre embryos. Each: t -test, * P ≤0.001, s.e.m. ; n =3 per genotype. Full size image Knockdown of endothelial Cdk5 leads to lymphatic dysfunction EC-specific Cdk5 knockout embryos exhibited markedly dilated vessels that were of lymphatic origin as they expressed Lyve1, but contained blood cells, demonstrating a persisting connection between lymphatic and blood vessels ( Fig. 2a and Supplementary Fig. 6a,b ). Also the primary lymph sacs of Cdk5 fl/fl Tie2Cre embryos were severely dilated and filled with blood ( Fig. 2b–d ). Moreover, lymphatic capillaries displayed defective patterning. They were covered with ectopic SMCs, irregularly dilated and showed decreased branching ( Fig. 2e–g ). 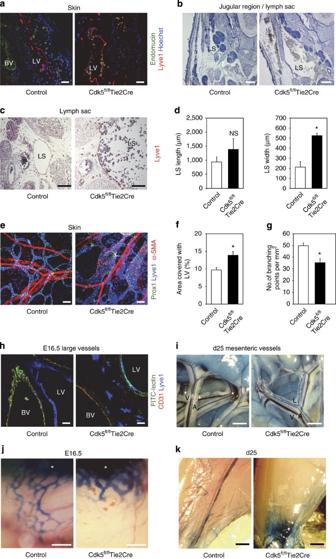Figure 2: Defective lymphatic vessel development in EC-specific Cdk5 deficient mice. (a) Lymphatic vessels (LVs) ofCdk5fl/flTie2Creembryos are dilated and contain blood cells. Staining of E16.5 transverse sections for endomucin (green, blood vessels), Lyve1 (red, LVs) and Hoechst 33342 (blue) show superficial vessels in the skin.n=5 per genotype. Scale bar, 20 μm. (b–d) Primary lymph sacs (LS) ofCdk5fl/flTie2Creembryos are dilated and filled with blood. (b) Haematoxylin/eosin (H/E) staining of E16.5 transverse sections at jugular regions. Scale bar, 200 μm. (c) Transverse sections at jugular regions of E16.5 embryos were stained for Lyve1 (red). Scale bar, 100 μm. (b,c)n=6 per genotype. (d) Quantification of LS length and width.t-test, *P≤0.05, s.e.m.n=3 per genotype. (e–g) Patterning defects and ectopic SMC coverage ofCdk5fl/flTie2CreLVs. (e) Whole-mount staining of E16.5 skin for Prox1 (green), Lyve1 (blue), α-SMA (red). Scale bar, 100 μm. (f) LV dilation ofCdk5fl/flTie2Creembryos indicated by an increased LV area. (g) Decreased LV branching ofCdk5fl/flTie2Creembryos. (f,g) Each:t-test, *P≤0.01, s.e.m.n=9 per genotype. (h) Abnormal connection between LVs and blood vessels (BVs) inCdk5fl/flTie2Creembryos. Intravenous injected FITC-lectin (green) exclusively stained BVs (CD31, red) of control embryos but labeled large collecting LVs (Lyve1, blue) inCdk5fl/flTie2Creembryos.n=3 per genotype. Scale bar, 20 μm. (i) Communication between lymphatic and blood vessels persisted in adult mice. Intravenous injected Evans blue dye exclusively labeled arteries (A) and veins (V) in control mice. InCdk5fl/flTie2Cremice, the dye also reached collecting mesenteric LVs (L).n=3 per genotype. Age: d20–25. Scale bar, 2 mm. (j,k) Impaired LV draining function inCdk5fl/flTie2Cremice. (j) Subcutaneously injected Evans blue was not removed from the injection site (asterisks) in E16.5Cdk5fl/flTie2Creembryos.n=3 per genotype. Scale bar, 0.5 mm. (k) Subcutaneously injected Evans blue (hind paw) was not drained away from the injection site inCdk5fl/flTie2Cremice, but labels tortuous LVs.n=3 per genotype. Age: d20–25. Scale bar, 1 mm. Figure 2: Defective lymphatic vessel development in EC-specific Cdk5 deficient mice. ( a ) Lymphatic vessels (LVs) of Cdk5 fl/fl Tie2Cre embryos are dilated and contain blood cells. Staining of E16.5 transverse sections for endomucin (green, blood vessels), Lyve1 (red, LVs) and Hoechst 33342 (blue) show superficial vessels in the skin. n =5 per genotype. Scale bar, 20 μm. ( b – d ) Primary lymph sacs (LS) of Cdk5 fl/fl Tie2Cre embryos are dilated and filled with blood. ( b ) Haematoxylin/eosin (H/E) staining of E16.5 transverse sections at jugular regions. Scale bar, 200 μm. ( c ) Transverse sections at jugular regions of E16.5 embryos were stained for Lyve1 (red). Scale bar, 100 μm. ( b , c ) n =6 per genotype. ( d ) Quantification of LS length and width. t -test, * P ≤0.05, s.e.m. n =3 per genotype. ( e – g ) Patterning defects and ectopic SMC coverage of Cdk5 fl/fl Tie2Cre LVs. ( e ) Whole-mount staining of E16.5 skin for Prox1 (green), Lyve1 (blue), α-SMA (red). Scale bar, 100 μm. ( f ) LV dilation of Cdk5 fl/fl Tie2Cre embryos indicated by an increased LV area. ( g ) Decreased LV branching of Cdk5 fl/fl Tie2Cre embryos. ( f , g ) Each: t -test, * P ≤0.01, s.e.m. n =9 per genotype. ( h ) Abnormal connection between LVs and blood vessels (BVs) in Cdk5 fl/fl Tie2Cre embryos. Intravenous injected FITC-lectin (green) exclusively stained BVs (CD31, red) of control embryos but labeled large collecting LVs (Lyve1, blue) in Cdk5 fl/fl Tie2Cre embryos. n =3 per genotype. Scale bar, 20 μm. ( i ) Communication between lymphatic and blood vessels persisted in adult mice. Intravenous injected Evans blue dye exclusively labeled arteries (A) and veins (V) in control mice. In Cdk5 fl/fl Tie2Cre mice, the dye also reached collecting mesenteric LVs (L). n =3 per genotype. Age: d20–25. Scale bar, 2 mm. ( j , k ) Impaired LV draining function in Cdk5 fl/fl Tie2Cre mice. ( j ) Subcutaneously injected Evans blue was not removed from the injection site (asterisks) in E16.5 Cdk5 fl/fl Tie2Cre embryos. n =3 per genotype. Scale bar, 0.5 mm. ( k ) Subcutaneously injected Evans blue (hind paw) was not drained away from the injection site in Cdk5 fl/fl Tie2Cre mice, but labels tortuous LVs. n =3 per genotype. Age: d20–25. Scale bar, 1 mm. Full size image As Cdk5 is ubiquitously expressed throughout the vasculature ( Supplementary Figs 1 and 3 ), and our own previous studies indicated functions of Cdk5 in blood vessel endothelial cells in vitro [19] , [20] , [21] , we checked whether blood vessels were affected by endothelial Cdk5 knockdown. Although knockdown of Cdk5 by the Tie2Cre driver resulted in Cdk5 downregulation in both lymphatic as well as blood endothelial cells ( Fig. 1i,j ), in contrast to the striking lymphatic vessel defects, blood vessel morphology of Cdk5 fl/fl Tie2Cre embryos was not affected. EphrinB2 and EphB4 were expressed at comparable levels in arteries and veins of control and Cdk5 fl/fl Tie2Cre embryos and SMC coverage of blood vessels was not changed ( Supplementary Fig. 5 ). This points to a specific function of Cdk5 in the lymphatic vasculature, like many genes that exert a tissue specific role, despite showing a wide expression pattern, for example, Rb for retinoblastoma [22] or Pkd1 for lymphatic vasculature [23] , [24] . In consequence, our further studies focused on the lymphatic vessel phenotype of EC-specific Cdk5 knockout mice. FITC-lectin or Evans Blue was intravenously injected to study the abnormal connection of blood and lymphatic systems. The dye exclusively stained blood vessels in control, but reached large collecting lymphatic vessels in Cdk5 fl/fl Tie2Cre mice ( Fig. 2h,i and Supplementary Fig. 6c ). FITC-lectin or Evans blue dye did not stain subcutaneous tortuous lymphatic microvessels of Cdk5 fl/fl Tie2Cre embryos ( Supplementary Fig. 6d,e ) indicating that the abnormal communication was not due to anastomosis between blood and lymphatic capillaries. The functionality of lymphatic vessels was further tested by subcutaneous injection of Evans blue at E16.5 or postnatally. The significantly impaired dye removal in Cdk5 fl/fl Tie2Cre mice demonstrated a lymphatic drainage defect ( Fig. 2j,k ). Lymphatic valve formation is arrested by Cdk5 knockout To understand the lymphatic drainage defect, we first analysed EC apoptosis, which was not affected in Cdk5 fl/fl Tie2Cre embryos ( Supplementary Fig. 7a–d ). Intraluminal valves are crucial for lymphatic function, and expressed Cdk5 ( Fig. 3a ). Stainings of skin and mesentery revealed reduced numbers of lymphatic valves and impaired lymphatic valve morphogenesis in EC-specific Cdk5 knockout embryos ( Fig. 3b–i and Supplementary Fig. 9 ). The majority of lymphatic valve forming cells failed to reorient and form valve leaflets ( Fig. 3f–i ), which was especially prevalent in embryos with severe phenotypes. Moreover, quantification of Prox1 positive nuclei of lymphatic endothelial cells pointed to hyperplasia of lymphatic vessels in Cdk5 fl/fl Tie2Cre embryos ( Supplementary Fig. 7e–h ). However, Cdk5 silencing ( Supplementary Fig. 8d ) influenced neither proliferation nor cell cycle of LECs ( Supplementary Fig. 8a,b ). Moreover, LEC cell size was not altered by Cdk5 knockdown ( Supplementary Fig. 8c ). Thus, lymphatic vessel hyperplasia seems not to be the major phenotype of endothelial-specific Cdk5 knockout mice. Therefore, our further studies focused on analysis of the lymphatic valve phenotype. We analysed whether the role of Cdk5 in lymphatic valve formation also encompasses lymphovenous valves, which separate the primordial thoracic duct (pTD) and adjacent cardinal vein (CV) [3] , [4] , [25] , [26] . Three-dimensional reconstructions of image stacks obtained by optical sectioning of entire whole-mount immunostained E12.5 embryos showed lymphovenous valves, that is, two contact sites of double layer of endothelial cells with high Prox1 expression, in control littermates and demonstrated frequent failure of lymphovenous valve formation in Cdk5 fl/fl Tie2Cre embryos ( Fig. 4 ). To understand whether Cdk5 is also essential for valve maintenance, we postnatally deleted endothelial Cdk5 in mature valves by using tamoxifen-inducible Cdh5(PAC)-CreERT2 mice. Lymphatic vessels and valves appeared normal in tamoxifen-treated Cdk5 fl/fl VECCre mice ( Fig. 5a,b ). In sum, our data demonstrate an indispensable endothelial cell autonomous requirement of Cdk5 for lymphatic vessel development and valve formation but not for valve maintenance. 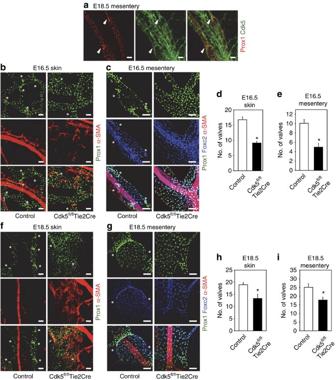Figure 3: Defective lymphatic valve formation in EC-specific Cdk5 knockout embryos. (a) Cdk5 expression in lymphatic valves. Whole-mount stainings of E18.5 mesenteric vessels show co-localization of Cdk5 (green) and Prox1 (red) (arrowheads).n=3. Scale bar, 50 μm. (b–e) Cdk5 controls lymphatic valve formation. Stainings of (b) skin and (c) mesenteric vessels of E16.5 embryos for Prox1 (green), Foxc2 (blue) and α-SMA (red). Valves are indicated by asterisks.n=9 per genotype. Scale bar, 50 μm. (d,e) Quantification of valves in E16.5 embryos.n=9 per genotype. (d) skin;t-test, *P≤0.001, s.e.m. (e) mesenteric vessels;t-test, *P≤0.001, s.e.m. (f–i) Cdk5 controls lymphatic valve maturation. Stainings of (f) skin and (g) mesenteric vessels of E18.5 embryos for Prox1 (green), Foxc2 (blue) and α-SMA (red). Valves are indicated by asterisks.n=5 per genotype. Scale bar, 50 μm. (h,i) Quantification of valves in E18.5 embryos. (h) Skin;t-test, *P≤0.05, s.e.m. (i) Mesenteric vessels;t-test, *P≤0.05, s.e.m; (h,i)n=5 per genotype. Figure 3: Defective lymphatic valve formation in EC-specific Cdk5 knockout embryos. ( a ) Cdk5 expression in lymphatic valves. Whole-mount stainings of E18.5 mesenteric vessels show co-localization of Cdk5 (green) and Prox1 (red) (arrowheads). n =3. Scale bar, 50 μm. ( b – e ) Cdk5 controls lymphatic valve formation. Stainings of ( b ) skin and ( c ) mesenteric vessels of E16.5 embryos for Prox1 (green), Foxc2 (blue) and α-SMA (red). Valves are indicated by asterisks. n =9 per genotype. Scale bar, 50 μm. ( d , e ) Quantification of valves in E16.5 embryos. n =9 per genotype. ( d ) skin; t -test, * P ≤0.001, s.e.m. ( e ) mesenteric vessels; t -test, * P ≤0.001, s.e.m. ( f – i ) Cdk5 controls lymphatic valve maturation. Stainings of ( f ) skin and ( g ) mesenteric vessels of E18.5 embryos for Prox1 (green), Foxc2 (blue) and α-SMA (red). Valves are indicated by asterisks. n =5 per genotype. Scale bar, 50 μm. ( h , i ) Quantification of valves in E18.5 embryos. ( h ) Skin; t -test, * P ≤0.05, s.e.m. ( i ) Mesenteric vessels; t -test, * P ≤0.05, s.e.m; ( h , i ) n =5 per genotype. 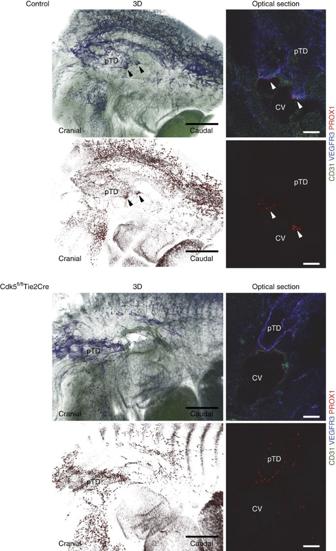Figure 4: Impaired lymphovenous valve formation in Cdk5 knockout embryos. Sagittal views of control andCdk5fl/flTie2Creembryos (E12.5) whole-mount immunostained for CD31 (green), VEGFR3 (blue) and Prox1 (red) are shown (left panels). Two contact sites between pTD and CV that express high levels of Prox1 indicate lymphovenous valves (arrowheads). Scale bar, 500 μm. Individual optical sections (right panels) through the contact area of pTD and CV are shown. In the control, two areas with a double layer of endothelial cells that express high levels of Prox1 indicate lymphovenous valves (arrowheads). Scale bar, 100 μm. Control:n=4. Three out of five analysedCdk5fl/flTie2Creembryos showed defects in lymphovenous valve formation. Full size image Figure 4: Impaired lymphovenous valve formation in Cdk5 knockout embryos. Sagittal views of control and Cdk5 fl/fl Tie2Cre embryos (E12.5) whole-mount immunostained for CD31 (green), VEGFR3 (blue) and Prox1 (red) are shown (left panels). Two contact sites between pTD and CV that express high levels of Prox1 indicate lymphovenous valves (arrowheads). Scale bar, 500 μm. Individual optical sections (right panels) through the contact area of pTD and CV are shown. In the control, two areas with a double layer of endothelial cells that express high levels of Prox1 indicate lymphovenous valves (arrowheads). Scale bar, 100 μm. Control: n =4. Three out of five analysed Cdk5 fl/fl Tie2Cre embryos showed defects in lymphovenous valve formation. 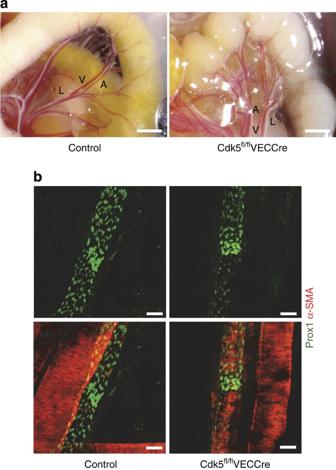Figure 5: Cdk5 is not essential for valve maintenance. (a) Normal lymphatic vessels in postnatally induced endothelial Cdk5 knockout mice. Mesentery of d10 control andCdk5fl/flVECCrepups treated with tamoxifen (d1–d3). Lymphatic vessel (L), artery (A) and vein (V) are indicated.n=2 per genotype. Scale bar, 2 mm. (b) Normal lymphatic valves in postnatally induced endothelial Cdk5 knockout mice. Staining of mesentery of d10 control andCdk5fl/flVECCrepups for Prox1 (green) and α-SMA (red).n=2 per genotype. Scale bar, 50 μm. Full size image Figure 5: Cdk5 is not essential for valve maintenance. ( a ) Normal lymphatic vessels in postnatally induced endothelial Cdk5 knockout mice. Mesentery of d10 control and Cdk5 fl/fl VECCre pups treated with tamoxifen (d1–d3). Lymphatic vessel (L), artery (A) and vein (V) are indicated. n =2 per genotype. Scale bar, 2 mm. ( b ) Normal lymphatic valves in postnatally induced endothelial Cdk5 knockout mice. Staining of mesentery of d10 control and Cdk5 fl/fl VECCre pups for Prox1 (green) and α-SMA (red). n =2 per genotype. Scale bar, 50 μm. Full size image Cdk5 controls Foxc2 activity by phosphorylation Next, we aimed to understand Cdk5-driven signaling in the lymphatic vasculature. We analysed expression of crucial LEC-specific genes whose inactivation or mutation revealed lymphatic vessel phenotypes reminiscent to endothelial Cdk5 knockout embryos: the forkhead transcription factor Foxc2 (ref. 10 ), the O-glycoprotein podoplanin [27] , [28] , T-synthase (T-Syn), that is, a glycosyltransferase critical for the biosynthesis of O-glycans including podoplanin [29] , the homeobox transcription factor Prox1 (ref. 4 ), Ets transcription factors Ets1 and Ets2 (ref. 30 ). The transcription factors Ets1, Ets2 and Foxc2 are regulated by phosphorylation at serine/threonine residues [30] , [31] and therefore might be of special interest as potential Cdk5 targets. However, we did not find obvious changes in expression of Foxc2, Prox1, Ets1 and Ets2, podoplanin or VEGFR3 ( Supplementary Fig. 10 ). Nevertheless, the defects of Cdk5 fl/fl Tie2Cre mice—defective lymphatic vessel patterning with ectopic SMC coverage, arrested valve formation, lymphatic dysfunction and lymphedema—are in striking similarity to Foxc2 deficient mice [10] . Foxc2 is a forkhead transcription factor crucial for lymphatic vessel development and valve formation [10] , [32] and is associated with human lymphedema-distichiasis [33] , [34] . In addition to lymphatic vessel defects, Foxc2-deficient mice show defects of aortic arch formation and skeletogenesis as well as cardiovascular defects. Foxc2−/− mice die within 10 min after birth due to respiratory defects and cyanosis, showing overall embryonic and perinatal lethality [35] , [36] . Thus, nevertheless, we hypothesized that Foxc2 could be the target of Cdk5 mediating its effects in the lymphatic endothelium. Therefore, we analysed the phenotype of Foxc2 knockout embryos. In fact, Foxc2−/− embryos (E13.5) showed edema formation and blood-filled lymphatic vessels, demonstrating that phenotypes of endothelial Cdk5 knockout and Foxc2-deficient embryos are similar ( Fig. 6 ). Foxc2 expression and electrophoretic mobility was not changed in LECs or BECs from EC-specific Cdk5 knockdown embryos ( Supplementary Fig. 11a–d,i ). As Foxc2 is expressed in multiple tissues, even small contamination in the LECs could significantly affect the results of the electrophoretic mobility assay. Therefore, we analyzed the electrophoretic mobility of Foxc2 in global Cdk5 knock-out embryos. Similar expression levels of Foxc2 in wild-type and global Cdk5 knockout embryos ( Supplementary Fig. 11j ) excluded that the unchanged electrophoretic mobility was due to EC contamination with other cells. In line, Cdk5 silencing in human LECs (hLECs) or HUVECs only slightly reduced Foxc2 ( Supplementary Fig. 11e–h,k,l ). Furthermore, Cdk5 downregulation did not influence Foxc2 localization ( Supplementary Fig. 11m ), nor Foxc2 binding to naked DNA ( Supplementary Fig. 12a,b ). However, Cdk5 overexpression ( Supplementary Fig. 12c ) significantly increased Foxc2 reporter gene activation ( Fig. 7a ), suggesting that Cdk5 is required for Foxc2 transcriptional activity. 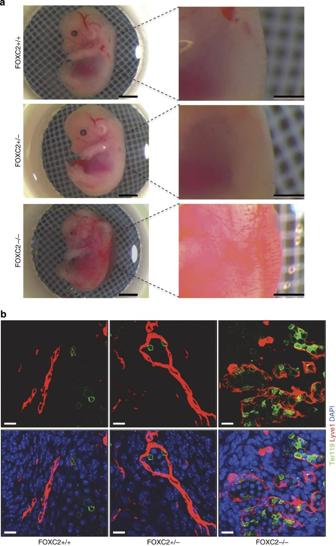Figure 6: Phenotypes of endothelial Cdk5 and Foxc2 knockout embryos are similar. (a) Blood-filled superficial capillaries, bleeding and edema formation in Foxc2 knockout embryos (Foxc2−/−, E13.5) are shown. Representative images ofFoxc2+/+(n=1),Foxc2+/−(n=6) andFoxc2−/−(n=6 withn=4 with obvious phenotype) littermates are shown. Scale bar, 2 mm at left panels. Scale bar, 1 mm at right panels. (b) Immunostainings reveal blood-filled lymphatic vessels inFoxc2−/−embryos. Lyve1 (red) indicates lymphatic vessels. Blood cells are stained by Ter119 (green). Scale bar, 10 μm. Figure 6: Phenotypes of endothelial Cdk5 and Foxc2 knockout embryos are similar. ( a ) Blood-filled superficial capillaries, bleeding and edema formation in Foxc2 knockout embryos ( Foxc2−/− , E13.5) are shown. Representative images of Foxc2+/+ ( n =1), Foxc2+/− ( n =6) and Foxc2−/− ( n =6 with n =4 with obvious phenotype) littermates are shown. Scale bar, 2 mm at left panels. Scale bar, 1 mm at right panels. ( b ) Immunostainings reveal blood-filled lymphatic vessels in Foxc2−/− embryos. Lyve1 (red) indicates lymphatic vessels. Blood cells are stained by Ter119 (green). Scale bar, 10 μm. 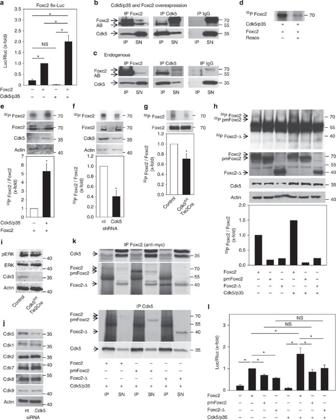Figure 7: Cdk5 controls Foxc2 by phosphorylation. (a) Cdk5 activates the Foxc2 luciferase reporter. Foxc2 reporter activity was analysed after co-transfection of HepG2 cells with empty vector, Foxc2, Cdk5/p35 or Foxc2 and Cdk5/p35. One-way analysis of variance (ANOVA; Student–Newman–Keuls) *P<0.05, s.e.m.n=5. (b,c) Interaction of Cdk5 and Foxc2. Immunoprecipitations of Foxc2, Cdk5 and IgG of (b) hLECs overexpressing Foxc2 and Cdk5/p35 or (c) untreated hLECs.n=3. IP, immunoprecipitation; SN, supernatant. (d) Cdk5 phosphorylates Foxc2in vitro. Recombinant Foxc2 and Cdk5/p35 were incubated with32P-ATP with/without the Cdk5 inhibitor roscovitine (rosco, 100 μM). SDS–PAGE and autoradiography were performed.n=2. (e–g) Cdk5 phosphorylates Foxc2in vivo. (e) Cdk5 overexpression increases Foxc232P incorporation. HUVECs overexpressing Foxc2 with/without Cdk5/p35.t-test, *P<0.01, s.e.m.n=3. (f) Cdk5 downregulation decreases Foxc232P incorporation. HUVECs transduced with non-targeting (nt) or Cdk5 shRNA and transfected with Foxc2.t-test, *P<0.05, s.e.m.n=2. (g) Foxc232P incorporation in E16.5 control andCdk5fl/flTie2CreLECs.t-test, *P<0.05, s.e.m.,n=3 per genotype. (h)32P incorporation into Foxc2-wt (Foxc2) and Foxc2 phosphorylation mutants Foxc2-A8 (pmFoxc2), or Foxc2-mutΔS219–366 (Foxc2-Δ) in the absence or presence of Cdk5 (Cdk5/p35) is shown.n=2. (i) Phosphorylated ERK (pERK) and ERK are not changed in E16.5Cdk5fl/flTie2CreLECs.n=2 per genotype. (j) Levels of Cdks1, 2, 7, 8, 9 are not changed by Cdk5 silencing in hLECs. (k) Interaction of Cdk5 with Foxc2 and Foxc2 phosphorylation mutants. Immunoprecipitations of Cdk5 and Foxc2 from HepG2 cells overexpressing Cdk5/p35 together with either Foxc2, pmFoxc2 or Foxc2-mutΔS219–366 were performed. Cdk5 coprecipitates with Foxc2 and pmFoxc2, and Foxc2-mutΔS219–366.n=3. IP, immunoprecipitation; SN, supernatant. (l) Cdk5-mediated phosphorylation controls Foxc2 transcriptional activity. Foxc2 reporter gene activity was analysed after co-transfection of HepG2 cells with empty vector, Foxc2, pmFoxc2 or Foxc2-mutΔS219–366 (Foxc2-Δ), with/without Cdk5/p35. Cdk5 induces Foxc2 reporter activation when co-expressed with Foxc2. When co-transfected with Foxc2 phosphorylation mutants pmFoxc2 or Foxc2-Δ, Cdk5 did not induce Foxc2 reporter activation. One-way ANOVA (Holm–Sidak) *P<0.001, s.e.m.n=4; NS, not significant. Full size image Figure 7: Cdk5 controls Foxc2 by phosphorylation. ( a ) Cdk5 activates the Foxc2 luciferase reporter. Foxc2 reporter activity was analysed after co-transfection of HepG2 cells with empty vector, Foxc2, Cdk5/p35 or Foxc2 and Cdk5/p35. One-way analysis of variance (ANOVA; Student–Newman–Keuls) * P <0.05, s.e.m. n =5. ( b , c ) Interaction of Cdk5 and Foxc2. Immunoprecipitations of Foxc2, Cdk5 and IgG of ( b ) hLECs overexpressing Foxc2 and Cdk5/p35 or ( c ) untreated hLECs. n =3. IP, immunoprecipitation; SN, supernatant. ( d ) Cdk5 phosphorylates Foxc2 in vitro . Recombinant Foxc2 and Cdk5/p35 were incubated with 32 P-ATP with/without the Cdk5 inhibitor roscovitine (rosco, 100 μM). SDS–PAGE and autoradiography were performed. n =2. ( e – g ) Cdk5 phosphorylates Foxc2 in vivo . ( e ) Cdk5 overexpression increases Foxc2 32 P incorporation. HUVECs overexpressing Foxc2 with/without Cdk5/p35. t -test, * P <0.01, s.e.m. n =3. ( f ) Cdk5 downregulation decreases Foxc2 32 P incorporation. HUVECs transduced with non-targeting (nt) or Cdk5 shRNA and transfected with Foxc2. t -test, * P <0.05, s.e.m. n =2. ( g ) Foxc2 32 P incorporation in E16.5 control and Cdk5 fl/fl Tie2Cre LECs. t -test, * P <0.05, s.e.m., n =3 per genotype. ( h ) 32 P incorporation into Foxc2-wt (Foxc2) and Foxc2 phosphorylation mutants Foxc2-A8 (pmFoxc2), or Foxc2-mutΔS219–366 (Foxc2-Δ) in the absence or presence of Cdk5 (Cdk5/p35) is shown. n =2. ( i ) Phosphorylated ERK (pERK) and ERK are not changed in E16.5 Cdk5 fl/fl Tie2Cre LECs. n =2 per genotype. ( j ) Levels of Cdks1, 2, 7, 8, 9 are not changed by Cdk5 silencing in hLECs. ( k ) Interaction of Cdk5 with Foxc2 and Foxc2 phosphorylation mutants. Immunoprecipitations of Cdk5 and Foxc2 from HepG2 cells overexpressing Cdk5/p35 together with either Foxc2, pmFoxc2 or Foxc2-mutΔS219–366 were performed. Cdk5 coprecipitates with Foxc2 and pmFoxc2, and Foxc2-mutΔS219–366. n =3. IP, immunoprecipitation; SN, supernatant. ( l ) Cdk5-mediated phosphorylation controls Foxc2 transcriptional activity. Foxc2 reporter gene activity was analysed after co-transfection of HepG2 cells with empty vector, Foxc2, pmFoxc2 or Foxc2-mutΔS219–366 (Foxc2-Δ), with/without Cdk5/p35. Cdk5 induces Foxc2 reporter activation when co-expressed with Foxc2. When co-transfected with Foxc2 phosphorylation mutants pmFoxc2 or Foxc2-Δ, Cdk5 did not induce Foxc2 reporter activation. One-way ANOVA (Holm–Sidak) * P <0.001, s.e.m. n =4; NS, not significant. Full size image Next, we wanted to understand how Cdk5 regulates Foxc2 activity. Recently, it has been shown that Foxc2 is phosphorylated at eight conserved serine/threonine residues, essential for Foxc2-dependent transcription but a kinase that mediates Foxc2 phosphorylation in vivo has not been identified yet [31] . Co-immunoprecipitation of overexpressed or endogenous Cdk5 and Foxc2 indicated their direct interaction in human LECs ( Fig. 7b,c ). In fact, we found that recombinant Cdk5/p35 efficiently phosphorylated Foxc2 in vitro , which was reduced by the Cdk5 inhibitor roscovitine ( Fig. 7d ). Arguing that Foxc2 is a direct substrate of Cdk5, Cdk5 overexpression increased 32 P-phosphate incorporation into Foxc2 ( Fig. 7e ), whereas Cdk5 silencing reduced 32 P-labelled Foxc2 ( Fig. 7f ). Importantly, Foxc2 32 P-phosphate incorporation was reduced in Cdk5 fl/fl Tie2Cre LECs in vivo ( Fig. 7g ). In line, Cdk5-mediated 32 P-phosphate incorporation was reduced in Foxc2 phosphorylation mutants (pmFoxc2: Foxc2-A8 with all eight serine/threonine residues mutated to alanine and Foxc2-Δ: Foxc2-mutΔS219–366 that lacks the complete phosphorylation region) ( Fig. 7h ). Thus, in sum, our data indicate that Cdk5 phosphorylates Foxc2. Interestingly, Cdk5 downregulation failed to induce a change in Foxc2 electrophoretic mobility ( Supplementary Fig. 11i–l ), characteristic for loss of Foxc2 phosphorylation [31] . This suggests that Cdk5 does not regulate all but only specific Foxc2 phosphorylation site(s). Moreover, this indicates that Foxc2 most likely gets regulated by additional other kinases besides Cdk5, that is, ERK1/2 and cell cycle Cdks, as it was previously suggested [31] . We checked whether Cdk5 collaborates with these pathways that have been associated with Foxc2 regulation, that is, ERK1/2 and cell cycle-related Cdks [31] . In Cdk5 fl/fl Tie2Cre LECs, neither ERK1/2 activity or expression ( Fig. 7i ) nor levels of cell cycle-related Cdks 1, 2, 7, 8, and 9 ( Fig. 7j ) were changed. This suggests that Cdk5 does not cooperate with these pathways in regulating Foxc2. We finally aimed to assess the functional relevance of Cdk5-mediated Foxc2 phosphorylation. Although Cdk5 alone did not activate the Foxc2 reporter, Cdk5 significantly increased wild-type Foxc2-driven reporter activation, that is, the Cdk5-mediated increase of Foxc2 reporter activation significantly differed from the effect of Foxc2-wt alone ( Fig. 7a,l ). In contrast, if Cdk5 was co-expressed with Foxc2 phosphorylation mutants—pmFoxc2: Foxc2-A8 with all eight serine/threonine residues mutated to alanine and Foxc2-Δ: Foxc2-mutΔS219–366 that lacks the complete phosphorylation region ( Supplementary Fig. 12d )—Cdk5 was not able to induce Foxc2 reporter activation, that is, there was no significant difference between the Foxc2 mutants with and without Cdk5 in Foxc2 reporter activation ( Fig. 7l ). Finally, immunoprecipitation experiments revealed that Cdk5 still interacts with the Foxc2 phosphorylation mutants Foxc2-A8 and Foxc2- mutΔS219–366 ( Fig. 7k ). A possible explanation is that Cdk5 might first interact with unphosphorylated Foxc2 and then add phosphate to the protein. Our data suggest that Cdk5 physically interacts with Foxc2. In summary, Cdk5 seems to be an upstream kinase of Foxc2 and to affect its phosphorylation status and transcriptional activity. Cdk5 regulates Foxc2 downstream target expression Disruption in Cdk5-Foxc2 signalling should affect Foxc2 target gene expression. Connexin37 (Cx37) is a downstream target of Foxc2 important for lymphatic valve formation [37] , [38] . Similar to Foxc2−/− mice, Cdk5 fl/fl Tie2Cre mice demonstrated attenuated Cx37 expression in lymphatic vessels, but not arteries ( Fig. 8a ). In line, quantitative PCR with reverse transcription (RT–PCR) analysis revealed more than 95% downregulation of Cx37 mRNA in Cdk5 fl/fl Tie2Cre LECs but not BECs ( Fig. 8b,c ). Moreover, Cdk5 silencing decreased Cx37 mRNA and protein in hLECs ( Fig. 8d,e ). Since induction of Cx37 requires oscillatory shear stress (OSS) in cultured LECs—mimicking lymphatic valve-forming characteristics in vivo [37] —we analysed whether Cdk5 affects Cx37 expression under OSS as well. Indeed, Cdk5 silencing resulted in reduced Cx37 in LECs that were cultivated under OSS ( Fig. 8f ), corroborating that Cdk5 is linked with the Foxc2–Cx37 pathway. Prox1 and VE-cadherin were analysed as markers and confirm LEC and BEC identity ( Supplementary Fig. 12e–h ). 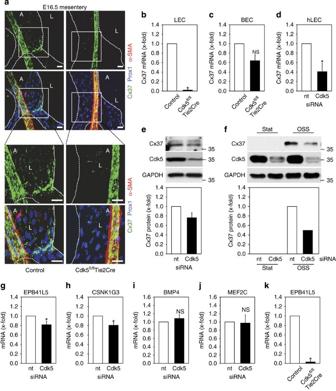Figure 8: Cdk5 regulates Foxc2 downstream target expression. (a) The Foxc2 downstream target connexin37 (Cx37) is decreased in LVs (L) but not arteries (A) ofCdk5fl/flTie2Creembryos. Whole-mount stainings of E16.5 mesentery for Cx37 (green), Prox1 (blue) and α-SMA. Lower panels show high magnification pictures.n=4 per genotype. Scale bar, 20 μm. (b,c) Cx37 mRNA is significantly decreased in (b)Cdk5fl/flTie2CreLECs but not (c) BECs.t-test, *P≤0.001, s.e.m.n=5 per genotype. (d) Cdk5 silencing decreases Cx37 mRNA in hLECs.t-test, *P≤0.05, s.e.m.n=4. (e) Cdk5 silencing decreases Cx37 protein in hLECs.n=2. (f) Cdk5 silencing decreases Cx37 protein in hLECs that was induced by oscillatory flow conditions (OSS). Immunoblots from hLECs treated with non-targeting (nt) or Cdk5 siRNA under OSS and detected with anti-Cx37, anti-Cdk5 and anti-GAPDH antibodies are shown. One representative experiment is displayed. (g,h) Expression of the Foxc2 downstream target genesEPB41L5andCSNK1G3is decreased in Cdk5 siRNA-treated hLECs. (g)EPB41L5:t-test, *P≤0.05, s.e.m.n=4. (h)CSNK1G3:t-test, *P≤0.05, s.e.m.n=5. (i,j) Expression of the Foxc2 downstream target genes (i)BMP4and (j)MEF2Cis not changed in Cdk5 siRNA treated hLECs. (i,j)t-test, NS, not significant, s.e.m., eachn=3. (k)EPB41L5mRNA is decreased in E16.5Cdk5fl/flTie2CreLECs.t-test, *P≤0.001, s.e.m.n=4 per genotype. Figure 8: Cdk5 regulates Foxc2 downstream target expression. ( a ) The Foxc2 downstream target connexin37 (Cx37) is decreased in LVs (L) but not arteries (A) of Cdk5 fl/fl Tie2Cre embryos. Whole-mount stainings of E16.5 mesentery for Cx37 (green), Prox1 (blue) and α-SMA. Lower panels show high magnification pictures. n =4 per genotype. Scale bar, 20 μm. ( b , c ) Cx37 mRNA is significantly decreased in ( b ) Cdk5 fl/fl Tie2Cre LECs but not ( c ) BECs. t -test, * P ≤0.001, s.e.m. n =5 per genotype. ( d ) Cdk5 silencing decreases Cx37 mRNA in hLECs. t -test, * P ≤0.05, s.e.m. n =4. ( e ) Cdk5 silencing decreases Cx37 protein in hLECs. n =2. ( f ) Cdk5 silencing decreases Cx37 protein in hLECs that was induced by oscillatory flow conditions (OSS). Immunoblots from hLECs treated with non-targeting (nt) or Cdk5 siRNA under OSS and detected with anti-Cx37, anti-Cdk5 and anti-GAPDH antibodies are shown. One representative experiment is displayed. ( g , h ) Expression of the Foxc2 downstream target genes EPB41L5 and CSNK1G3 is decreased in Cdk5 siRNA-treated hLECs. ( g ) EPB41L5 : t -test, * P ≤0.05, s.e.m. n =4. ( h ) CSNK1G3 : t -test, * P ≤0.05, s.e.m. n =5. ( i , j ) Expression of the Foxc2 downstream target genes ( i ) BMP4 and ( j ) MEF2C is not changed in Cdk5 siRNA treated hLECs. ( i , j ) t -test, NS, not significant, s.e.m., each n =3. ( k ) EPB41L5 mRNA is decreased in E16.5 Cdk5 fl/fl Tie2Cre LECs. t -test, * P ≤0.001, s.e.m. n =4 per genotype. Full size image Foxc2 phosphorylation was shown to selectively recruit Foxc2 to chromatin, differentially regulating expression of specific Foxc2 target genes [31] . Thus, next we aimed to clarify whether Cdk5-mediated activation of Foxc2-dependent transcription is due to phosphorylation. Therefore, we investigated the influence of Cdk5 on the expression of Foxc2 target genes that have been found to be dependent or independent on Foxc2 phosphorylation. Corroborating our previous results, Cdk5 silencing in hLECs decreased EPB41L5 and CSNK1G3 , Foxc2 downstream target genes that require Foxc2 phosphorylation [31] ( Fig. 8g,h ) but did not regulate BMP4 and MEF2C , Foxc2 target genes that do not depend on its phosphorylation [39] ( Fig. 8i,j ). Importantly, in vivo , EPB41L5 mRNA was reduced in Cdk5 fl/fl Tie2Cre LECs ( Fig. 8k ). Thus, Cdk5 specifically influences the expression of Foxc2 target genes that depend on Foxc2 phosphorylation, demonstrating that Cdk5 controls Foxc2-dependent transcription by phosphorylation. Foxc2 phosphorylation regulates its chromatin recruitment only in the context on native chromatin, but not in reconstituted in vitro systems [31] . Therefore, although Cdk5 did not influence Foxc2 binding to naked DNA ( Supplementary Fig. 12a,b ), our results raise questions regarding the role of Cdk5 in the interaction of Foxc2 with DNA and transcription-associated proteins. Taken together, our results demonstrate that Cdk5 is essential for lymphatic vessel development and valve formation. We highlight Cdk5 as an important player in the transcriptional control of lymphatic vessel remodelling, suggesting a function of Cdk5 in linking cell signalling and gene expression in the lymphatic endothelium. Our study provides the rationale for investigating CNS-related Cdk5-driven signalling in the context of lymphatic vessel biology with the aim to better understand the mechanism underlying human lymphedema syndromes. Endothelial-specific Cdk5 knockout mice Mouse experiments were performed with approval by the District Government of Upper Bavaria in accordance with the German animal welfare and institutional guidelines. Tie2Cre mice were from Jackson Laboratory ( B6.Cg-Tg(Tek-cre)12Flv/J , 004128). Floxed Cdk5 mice [40] , tamoxifen-inducible Cdh5(PAC)-CreERT2 mice [13] and deleterCre mice [41] were described. To obtain Cdk5 fl/fl Tie2Cre , Cdk5 fl/fl Cdh5(PAC) – CreERT2 (Cdk5 fl/fl VECCre) or Cdk5 fl/ Δ Tie2Cre mice, Cdk5 fl/fl or Cdk5 wt/ Δ females were crossed to Cdk5 wt/fl Tie2Cre or Cdk5 wt/fl VECCre males. To induce Cdk5 downregulation, pregnant mice were injected with tamoxifen (100 μl, 10 mg per ml in peanut oil) on E10.5, E11.5, E12.5 and embryos were collected at E16.5. Primers for genotyping: Cdk5 floxed: 5′-ctgcatttctcgtccctagc-3′; 5′-acgcttcagagccacaatct-3′. Cdk5 excised: 5′-ctgcatttctcgtccctagc-3′; 5′-ggccctgctttgtatctctg-3′. Tie2Cre: 5′-gctgccacgaccaagtgacagcaatg-3′; 5′-gtagttattcggatcatcagctacac-3′. Cdh5(PAC)-CreERT2 and deleterCre: 5′-gcctgcattaccggtcgatgcaacga-3′; 5′-gtggcagatggcgcggcaacaccatt-3′. Tracer experiments Evans blue (1% in PBS, E2129 Sigma) or FITC-lectin (1 mg ml −1 in PBS, L9381 Sigma) was injected intravenously (LV/BV separation; E16.5 embryos: periorbital sinus, 3 μl; anaesthesized adult mice: tail vein, 250 μl) or subcutaneously (LV function; E16.5 embryos 3 μl; anaesthesized adult mice: hind paw, 100 μl). Olympus SZX7/SZ-BI30 stereomicroscope, Olympus DP25 camera, CellSens software version 1.3. Immunohistochemistry For paraffin sections, tissues were fixed with 4% formalin for 24 h, left in 1%formalin, paraffin embedded and sectioned (5 μm). For cryosections, tissues were frozen into TissueTek. For Cdk5 stainings, embryos were frozen in liquid nitrogen directly after preparation, and frozen embryos were embedded into TissueTek. Ten-micrometre sections were prepared and fixed with formalin 4% (10 min, room temperature (RT)). Sections were blocked (1% BSA/PBS), incubated with primary antibodies (2 h RT or overnight (o/n) 4 °C), washed, incubated with AlexaFluor-labelled secondary antibodies (45 min, RT) and Hoechst 33342 (5 μg ml −1 ) or detection was performed using Vectastain ABC Kit and ImmPACT AEC Peroxidase Substrate Kit (Biozol) and mounted (Fluorsave Reagent, Calbiochem). For Cdk5 staining, the Vector M.O.M. (mouse on mouse) Immunodetection Kit was used according to manufacturer’s instructions. For TUNEL staining, ApopTag Plus Fluorescein In Situ Apoptosis Detection Kit (S7110, Millipore) was used. Liver: four mice, 60 fields; brain: four mice, 30 fields; spinal column: three mice, six fields per genotype. Proliferating Ki67-positive cells. E16.5: three mice, 36 pictures; E13.5: five mice, at least 47 pictures per genotype. Whole-mount stainings Tissues were fixed (formalin 4%, 30 min, RT or methanol 5 min, −20 °C), washed, blocked (1 h, RT, 0.5% TritonX, 2% BSA/PBS), incubated with primary antibodies (o/n, 4 °C), washed, incubated with AlexaFluor-labeled secondary antibodies (2 h, RT) and mounted. Valve analysis was done in back skin and intestines of E16.5 and E18.5 embryos [37] . E16.5: nine embryos; E18.5: five embryos per genotype. Numbers of valves were calculated in 10 fields (skin) or four mesenteric branches per embryo. Primary antibodies: CD31 (553370, BD Pharmingen), Cdk5 (AHZ0492, Life Technologies), Connexin37 (ref. 37 ), endomucin (sc-65495, Santa Cruz), EphB4 (AF446, R&D Systems), ephrinB2 (AF496, R&D Systems), Ets1 (sc-350, Santa Cruz), Ets2 (sc-351, Santa Cruz), Foxc2 (ref. 37 ), Ki67 (ab15580, Abcam), Lyve1 (ab14917, Abcam), p35 (sc-820 Santa Cruz), podoplanin (sc-134483, Santa Cruz), Prox1 (AF2727, R&D Systems), α-SMA (C6198, Sigma), Ter119 (14–5921, eBioscience), VEGFR3 (AF743, R&D Systems). Primary antibodies were used at 1:100 dilution. AlexaFluor-labelled secondary antibodies (Life Technologies) were used at 1:400 dilution. Pictures were taken with an Olympus BX41 microscope or with a Zeiss LSM 510 META confocal microscope. ImageJ and the particle counter plugin were used for counting. Lymphovenous valve staining Whole-mount staining of E12.5 embryos was performed as previously described [3] . In brief, embryos were fixed (2 h RT), permeabilized (0.5% TX in PBS, 4 °C, 48 h), blocked (1% BSA, 0.1% Tween20 in PBS, 4 °C, 48 h), incubated with primary antibodies (anti-Prox1, 102-PA32 Relia Tech; anti-CD31 553370 BD Biosciences; anti-VEGFR3, AF743 R&D Systems) in blocking solution (1:200, 4 °C, 1 week), washed (0.1% Tween in PBS, 2 days), incubated with secondary antibodies (AlexaFlour, Life Technologies, 1:1,000, 4 °C, 1 week) and washed (0.1% Tween in PBS, 2d) before clearing with BABB. Embryos were imaged using a Leica SP8 SMD confocal microscope with appropriate software. Isolation of mouse liver sinusoidal endothelial cells (LSECs) LSECs were isolated according to manufacturer’s instructions (Milteny Biotech miniMACS Separation System). Isolation of mouse LECs and BECs LECs and BECs were isolated from mouse embryo skin as described [37] , [42] with some modifications. In detail, the following protocol was used: Digestion . Embryonic skin was washed with DMEM with 20% FCS, digested (2.5 mg ml −1 Collagenase Type II, Worthington LS002140, 2.5 mg ml −1 Collagenase Type IV, Worthington LS004176, 1 mg ml −1 DNAse Type I Worthington LS004188, 1 mM β-glycerophosphate in DMEM; 1 ml per embryo; 37 °C, 30 min), passed through a cell strainer, centrifuged (1,200 g , 10 min, 4 °C) and resuspended in 10 ml HHF (5% FCS, 0.1 M HEPES in HBBS, Sigma H9394). Cells were counted and centrifuged (14,000 g , 5 min, 4 °C). Macrophage and leukocyte removal . Cells were resuspended in HHF (10 8 cells per ml maximum). F4/80 (CALTAG Labs MF48000) and CD45 antibodies (BD Pharmingen 553076; 10 μl each) were added. After gentle rotation (4 °C, 5 min), 15 volumes MACS buffer (0.5% BSA, 2 mM EDTA in PBS) were added, cells were centrifuged(1,400 g , 5 min, 4 °C), resuspended in MACS buffer (80 μl per 10 7 cells) Goat-anti-rat microbeads (Miltenyi Biotech 130-042-201; 20 μl per 107 cells) were added. After rotation (15 min, 4 °C), 15 volumes MACS buffer were added, cells were centrifuged (1,400 g , 5 min, 4 °C), resuspended (107 cells per 500 μl MACS buffer) and applied onto a pre-separation filter (Miltenyi Biotech 130-041-407) on a MS column (Miltenyi Biotech 130-042-201). After washing, (3 × 500 μl MACS buffer), flow-through containing LECs and BECs was collected. All the steps were repeated. Dead cell removal . Cells were resuspended in 100 μl Dead Cell Removal Microbeads (Milteny Biotech 130-090-101). After gentle rotation (RT, 15 min), 500 μl binding buffer was added, cells were applied onto a MS column, washed (4 × 500 μl binding buffer) and flow-through containing LECs and BECs was collected. LEC isolation . Cells were resuspended in HHF (10 8 ml −1 maximum). Lyve1 antibodies (AngioBio 11-034, 5 μl) were added. After gentle rotation (4 °C, 5 min), 15 volumes MACS buffer were added, cells were centrifuged (1,400 g , 5 min, 4 °C), resuspended in MACS buffer (80 μl per 10 7 cells). Goat-anti-rabbit microbeads (Miltenyi Biotech 130-048-602; 20 μl per 10 7 cells) were added. After rotation (15 min, 4 °C), 15 volumes of MACS buffer were added, cells were centrifuged (1,400 g , 5 min, 4 °C), resuspended (107 cells, 500 μl MACS buffer) and applied onto an MS column. After washing (3 × , 500 μl MACS buffer), flow-through containing BECs was collected. LECs were flushed out, and again applied to a separation column to increase LEC purity. BEC isolation . Cells were resuspended in HHF (10 8 per ml maximum). CD31 antibodies (BD Pharmingen 553370, 10 μl) were added. After gentle rotation (4 °C, 5 min), 15 volumes of MACS buffer (0.5% BSA, 2 mM EDTA in PBS) were added, cells were pelleted (1,400 g , 5 min, 4 °C), resuspended in MACS buffer (80 μl per 10 7 cells). Goat-anti-rat microbeads (20 μl per 10 7 cells) were added. After rotation (15 min, 4 °C), 15 volumes MACS buffer were added, cells were centrifuged (1,400 g , 5 min, 4 °C), resuspended (107 cells in 500 μl MACS buffer) and applied onto an MS column. After washing (3 × 500 μl MACS buffer), BECs were flushed out and again applied to a separation column to increase BEC purity. LECs and BECs were cultured on fibronectin (Roche 10838039001)-coated plates (24-well) with EGM2 (Lonza). Cell culture HUVECs (C-12253, PromoCell) were cultured as described [19] with endothelial cell growth medium (ECGM, C-22010 PromoCell) containing 10% FCS and penicillin/streptomycin. Human telomerase-immortalized LECs (hLECs, S. Geleff, University of Vienna, Vienna, Austria) [43] , [44] were cultivated in EGM2-MV (Lonza) and HepG2 cells (ACC-180, DSMZ) in DMEM with 10% FCS. Cell transfection The amaxa system (Lonza) with HUVEC nucleofector kit (VPB-1002, ECs) or cell line kit T (VCA-1002, HepG2) was used [19] . siRNAs (Dharmacon): ON-TARGETplus non-targeting (nt) siRNA D-001810-01-05; ON-TARGETplus Cdk5 siRNA J-003239-10 (5′-CCGGGAGACUCAUGAGAUC-3′) and J-003239-09 (5′-UAUAAGCCCUAUCCGAUGU-3′). Plasmids: Cdk5 (addgene 1871), p35 (addgene 1347), Foxc2 (ref. 39 ), Foxc2-mutA8 and Foxc2-mutΔ219–366 (ref. 31 ). Adenoviral transduction: Sirion Biotech GmbH (Martinsried, Germany). RT–PCR mRNA isolation was done with Qiagen RNeasy Mini Kit, reverse transcription with High-Capacity cDNA Reverse Transcription Kit (Applied Biosystems), and RT–PCR with the 7300 Real Time PCR System. Taqman gene expression assays: BMP4 Mm00432087_m1, connexin37 Hs00704917_s1 and Mm00433610_s1, Cdk5 Hs00358991_g1 and Mm01134945_g1, CSNK1G3 Mm00666283_m1, EPB41L5 Mm00521096_m1, Foxc2 Hs00270951_s1 and Mm00546194_s1, MEF2C Mm01340842_m1, Prox1 Hs00896294_m1 and Mm00435969_m1, VE-cadherin Mm00486938_m1 (Applied Biosystems). GAPDH was used as housekeeper. Shear stress experiments hLECs were transfected with Cdk5 or non-targeting siRNA, seeded at confluence on fibronectin-coated slides (μ-Slide I0.8 Luer; ibidi), cultured for 24 h and subjected to oscillatory flow (4 dynes cm −2 , ¼ Hz) in a parallel plate flow chamber system (ibidi Pump System; ibidi) or kept under static conditions for 48 h. At the end of the experiments, cell lysates were analysed by western blotting. Immunoblotting Immunoblotting was performed as described [19] . Primary antibodies (used at 1:1,000 dilution): actin (MAB 150 1R, Chemicon), Cdk1 (9116, Cell Signalling), Cdk2 (sc-163, Santa Cruz), Cdk5 (AHZ0492, Life Technologies), Cdk7 (2916, Cell Signalling), Cdk8 (sc-1521, Santa Cruz), Cdk9 (sc-13130, Santa Cruz), ERK (p44/p42 MAPK, 9202, Cell Signalling), ERK-phspho (p44/p42 MAPK, 9206, Cell Signalling), Ets1 (sc-350, Santa Cruz), Ets2 (sc-351, Santa Cruz), Foxc2 (AF5044, R&D Systems), Lyve1 (ab14917, R&D Systems), podoplanin (sc-134483, Santa Cruz), Prox1 (AF2727, R&D Systems), VEGFR3 (AF743, Abcam). Secondary antibodies (used at 1:1,000 dilution): goat anti mouse (BZL07046, Biozol), goat anti rabbit (172–1019,. Bio-Rad), donkey anti goat (2020, Santa Cruz), goat anti mouse (HAF007, R&D Systems). Full blots related to respective figures are shown in Supplementary Fig. 13 . Immunoprecipitation After cell lysis, anti-Cdk5 (5 μl per sample, AHZ0492, Life Technologies), anti-Foxc2 (5 μl per sample, AF5044, R&D Systems) or anti-myc (2.5 μl per sample, sc-40, Santa Cruz) antibodies were added with samples containing 200–500 μg protein. After incubation (o/n, 4 °C), ProteinG beads (50 μl per sample, P3296, Sigma) were added. After incubation (3 h, 4 °C), proteins were extracted and subjected to immunoblotting. Luciferase reporter assay HepG2 cells were transfected as indicated. Luciferase plasmids were 6xFOXC2-luc-reporter (firefly) [39] pGL4.74[hRluc/TK] (Renilla, Promega). Dual-Luciferase Reporter Assay System (Promega) and an Orion II Microplate Luminometer (Berthold) were used. Electrophoretic mobility shift assay Electrophoretic mobility shift assay (EMSA) was performed following a previously described protocol [45] . In detail, cells were scraped off in PBS, and nuclear extracts were prepared by incubation of cells in ice-cold buffer containing N-(2-hydroxyethyl)piperazine-N’-(2-ethanesulfonic acid; HEPES) pH 7.9 10 mM, KCl 10 mM, EDTA 0.1 mM, ethylene glycol-O,O’-bis-(2-amino-ethyl)-N,N,N’,N’,-tetraacetic acid (EGTA) 0.1 mM, dithio-1,4-threitol (DTT) 1 mM, PMSF 0.5 mM and Complete 1% for 15 min. Afterwards, Nonidet P-40 was added, the homogenate was vortexed and centrifuged. The nuclear pellet was resuspended by vigorous rocking for 15 min at 4 °C in a buffer containing HEPES pH 7.9 20 mM, NaCl 400 mM, EDTA 1 mM, EGTA 0.5 mM, glycerol 25%, DTT 1 mM, PMSF 1 mM and Complete 2%, centrifuged and the supernatant containing nuclear proteins was frozen at −80 °C. Equal amounts of nuclear proteins (2 μg) were incubated with radiolabelled Foxc2 oligonucleotides (1 μl, 5′-gatcccttaagtaaacagcatgagatc-3′, 5′-gatctcatgctgtttacttaagggatc-3′ (Biomers)) in a reaction buffer for 30 min and resolved by electrophoresis. Bands were visualized by applying the gels to Cyclone Storage Phosphor Screens (Canberra-Packard, Dreieich, Germany) and analysis by a phosphorimager (Cyclone Storage Phosphor System, Canberra-Packard, Dreieich, Germany). Kinase assay Recombinant Foxc2 (2.5 μg per sample, H00002303, Abnova) and Cdk5/p35 (20 ng per sample, 14–477, Millipore) were incubated with 32 P-ATP (10 μCi per sample, Hartmann Analytic) with/without roscovitine (100 μM, R7772, Sigma-Aldrich). SDS–PAGE and autoradiography were performed. Phosphate incorporation HUVECs, human LECs or HepG2 cells were transfected as indicated. Primary LECs were isolated from embryo skin. Eighteen hours after transfection or isolation, cells were incubated with 32 P orthophosphate (NEX053010MC, PerkinElmer) for 12 h in phosphate-free medium (DMEM, 11971, Gibco). Foxc2 immunoprecipitation, SDS–PAGE and autoradiography were performed. Statistics Numbers of independently performed experiments, the respective statistical test and the P value are indicated in the figure legends. Graph data represent means±s.e.m. Statistical analysis was performed using SigmaStat software Version 3.1. How to cite this article: Liebl, J. et al. Cdk5 controls lymphatic vessel development and function by phosphorylation of Foxc2. Nat. Commun. 6:7274 doi: 10.1038/ncomms8274 (2015).